The interplay between apparent viscosity and wettability in nanoconfined water Understanding and manipulating fluids at the nanoscale is a matter of growing scientific and technological interest. Here we show that the viscous shear forces in nanoconfined water can be orders of magnitudes larger than in bulk water if the confining surfaces are hydrophilic, whereas they greatly decrease when the surfaces are increasingly hydrophobic. This decrease of viscous forces is quantitatively explained with a simple model that includes the slip velocity at the water surface interface. The same effect is observed in the energy dissipated by a tip vibrating in water perpendicularly to a surface. Comparison of the experimental data with the model shows that interfacial viscous forces and compressive dissipation in nanoconfined water can decrease up to two orders of magnitude due to slippage. These results offer a new understanding of interfacial fluids, which can be used to control flow at the nanoscale. Crucial for the understanding of fluid flow in nanosize spaces is the liquid–solid interface [1] . Interfacial and nanoconfined liquid flow is relevant for biology [2] , [3] , tribology [4] , nanofluidics and high-resolution three-dimensional, two-dimensional printing [5] . Confined fluids exhibit unique structural, dynamical, electrokinetic and mechanical properties that are different from those of the bulk [6] , [7] , [8] , [9] , [10] . It is now well-known that liquids confined between surfaces, especially at gaps below a few nanometres, can present a dramatic increase in their viscosity [6] , [7] , [11] , [12] . Experiments and theory have shown that the viscosity of water confined between hydrophilic surfaces increases with confinement, reaching values orders of magnitude higher than bulk water when confined in a subnanometre gap [6] , [7] , [11] , [12] . It is also clear that the usual no-slip boundary condition, that is, zero fluid velocity at the motionless surface, is not universal, and experiments and computer simulations have proved that liquid molecules can slip and have a non-zero velocity at a still solid surface [13] , [14] , [15] . Furthermore, several studies have indicated that the amount of liquid slip strongly depends on the morphology and chemistry of the stationary solid surface [16] , [17] . However, no experiments have so far investigated the interrelationship between the viscosity of nanoconfined water, the wettability of the confining surfaces and the interface slippage. Here we present experiments using an atomic force microscope (AFM) showing that the interfacial viscous forces in nanoconfined water increase substantially for more hydrophilic confining surfaces, and for increasing confinement. We use a selection of atomically flat surfaces exhibiting different wetting properties and compare, as a function of confinement, viscous forces, energy dissipation and water slippage. This approach enables us to unambiguously single out the influence of surface properties (wetting) on the measured viscosity/dissipation. A comparison of the experimental data with a modified form of the Newtonian definition of viscosity that includes slippage demonstrates that the origin of this increase in viscous force (and apparent viscosity) is a reduced slippage at the surface. On the other hand, the intrinsic viscosity of nanoconfined water is not affected by surface hydrophilicity at any confinement size, until the last water layer close to the surface, and remains extremely high compared with that of bulk water. The same modified Newtonian model is then used to explain the dependence of energy dissipation on surface wettability in dynamic AFM experiments in water. For a given confinement size d , both the ratios of the viscous forces and energy dissipation measured on a variety of surfaces and on a surface with zero slip length b , are equal to d /( b + d ), as predicted by the definition of viscosity for a shear velocity gradient of v shear /( d + b ). These measurements reveal the relationship between water viscous interfacial forces and slippage, as well as the link between the nanoconfined water apparent viscosity and wettability. These results have important implications in nanotechnology and bionanoscience where the interaction in water between surfaces and objects at the nanoscale is mediated by the properties and the dynamic behaviour of water. AFM viscous force measurements By using an AFM, we have measured the shear viscous force, F shear , experienced in water by a nanosize AFM tip, while it is sheared parallel to an atomically smooth solid surface, as a function of the tip–surface distance, d (see Fig. 1a ). These viscous force curves, F shear ( d ), have been measured for five surfaces with different wettabilities, characterized by the static contact angle of water, θ (see inset of Fig. 2 , Supplementary Fig. S1 and Supplementary Table S1 ). We find a strong dependence of the viscous force on wettability, with force values varying from one surface to another one up to an order of magnitude at d ≈0.3 nm, corresponding approximately to one layer of water molecules on the solid surface. Viscous (shear) and solvation (normal) forces at the tip are measured simultaneously as a function of the tip–surface distance by detecting, respectively, the torsion and bending of a rectangular cantilever rigidly attached to the silicon tip, while it approaches a smooth solid surface in deionized ultra-filtered (DIUF) water (see Fig. 1 and Methods part). During the approach, the cantilever is laterally sheared by means of a lock-in amplifier with a shearing amplitude and frequency of 0.9 nm and 1 kHz, respectively. We remark that for this shearing speed, v shear =900 nm s −1 , the lateral force is mainly viscous, as measured from the 90° phase shift with the displacement [7] . The atomically smooth solid surfaces used in the viscosity measurements are, from the most to the least hydrophilic, on mica, graphene oxide (GO), silicon, diamond-like carbon (DLC), and highly oriented pyrolytic graphite (HOPG) (see Methods part for more details). The static contact angles have been characterized by imaging a small water droplet on the different surfaces ( Supplementary Fig. S1 ). A large contact angle indicates a poorly wetting surface, also referred as hydrophobic surface for the case of water, whereas vanishing contact angles indicate wetting surfaces, also called hydrophilic surfaces for water. 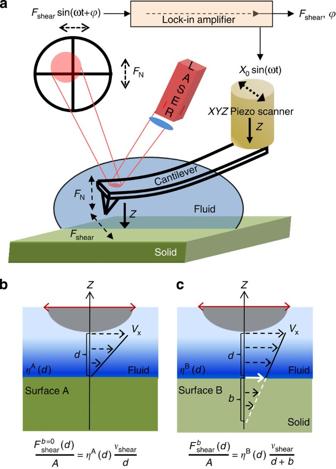Figure 1: The experimental setup and schematics of the boundary conditions. (a) Overview of the experimental setup. (b) Fluid velocity profile for a no-slip boundary condition (b=0) and for (c) a finite slip boundary condition (b≠0). The slip length is defined as the distance between the solid–fluid interface and the point where the velocity profile extrapolates to zero. Figure 1: The experimental setup and schematics of the boundary conditions. ( a ) Overview of the experimental setup. ( b ) Fluid velocity profile for a no-slip boundary condition ( b =0) and for ( c ) a finite slip boundary condition ( b ≠0). The slip length is defined as the distance between the solid–fluid interface and the point where the velocity profile extrapolates to zero. 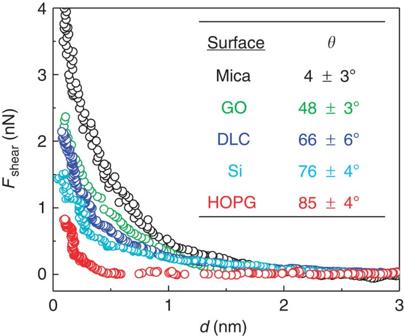Figure 2: Shear viscous force curves. The averaged shear viscous force curves encountered by shearing (νshear=900 nm s−1) a nanosize AFM tip in water when approaching solid surfaces with different wettabilities. Namely, mica (black), GO (green), DLC (blue), Si (cyan) and HOPG (red). The inset shows the measured contact angles on the respective surfaces. The viscous force data are averaged from multiple shear viscous force curves fromd=0.1 to 3 nm. SeeSupplementary Table S2for more details. Full size image Figure 2: Shear viscous force curves. The averaged shear viscous force curves encountered by shearing ( ν shear =900 nm s −1 ) a nanosize AFM tip in water when approaching solid surfaces with different wettabilities. Namely, mica (black), GO (green), DLC (blue), Si (cyan) and HOPG (red). The inset shows the measured contact angles on the respective surfaces. The viscous force data are averaged from multiple shear viscous force curves from d =0.1 to 3 nm. See Supplementary Table S2 for more details. Full size image Viscous forces as a function of surface wettability Figure 2 shows the shear viscous forces acting on an AFM tip when it approaches surfaces with different wettability in water as a function of the tip–surface separation. The calibration of the force–distance curve can be found in Supplementary Note 1 . For each surface, the curves are averaged over multiple force curves as described in the Supplementary Note 2 and Supplementary Table S2 . For all the investigated surfaces, the viscous force F shear approaches a value close to zero within the experimental error at d >3 nm and increases dramatically for d approaching zero. We remark that for larger distances the measured F shear is almost zero, because the viscosity of bulk water is too small to be measured with our instrument. On the other hand, when the tip is very close to the surface, d <2 nm, the increased F shear experienced by the tip at its apex is large enough to be detected as the torsion of the cantilever, as already reported in previous studies performed on mica [6] , [7] , [11] , [12] . Finally, much higher shear forces can be observed when the tip indents the solid’s surface. Nevertheless, although all the investigated solid surfaces give rise to a qualitatively similar trend in viscous forces, for fixed tip–surface distances the viscous force clearly decreases from mica to GO, DLC, Si and HOPG, respectively. To understand the origin of this decrease in the observed viscous force as a function of the interface material, we have characterized the wettability of the surfaces with static contact angle measurements. The static contact angles of water for the investigated surfaces are the following: θ Mica =4±3°, θ GO =48±3°, θ DLC =66±6°, θ Si =76±4° and θ HOPG =85±4°. As shown in Fig. 2 , larger viscous forces correlate with smaller contact angles (more hydrophilic/wetting surfaces). The observed relationship between contact angle and interfacial viscous force suggests that the interfacial slippage, which is known to often increase with the static contact angle of the surface [18] , may have a crucial role in the interfacial viscous forces. To demonstrate this hypothesis and to extract more quantitative information from these results, a modified Newtonian definition of viscosity is used for further analysis. A modified form of Newtonian viscosity and slip For a Newtonian fluid confined between two flat plates separated by a distance d , the shear force required to slide one plate parallel to a stationary one is proportional to the gradient of the fluid velocity in the direction perpendicular to the plates, ∂ v x /∂z (see Fig. 1b ): The proportionality factor, η , is defined as the viscosity of the liquid, whereas A is the area of the shearing plate. If the velocity profile is simply linear with no slippage, as shown in Fig. 1b , we have ∂ v x /∂z= v shear / d , where v shear is the shear velocity of the top plate. On the other hand, for a linear velocity profile with a finite slip length b as illustrated in Fig. 1c , we will have: As a first approximation, we can consider that the velocity profile of water between the AFM tip and the solid surface to be linear. Furthermore, for d <2 nm, the tip apex can be approximated to be a planar surface, as described in previous work [6] . Next we can combine equations (2) and (1) to obtain the ratio between the shear force in water close to surface B with b ≠0 and surface A with b =0 (see Fig. 1 ): where and are, respectively, the shear viscous force and the viscosity as a function of the tip–surface distance measured in water close to a surface with slip length equal to b . We note that in equation (3) the viscosity is a function of d , as it is known that for nanoconfined water the viscosity can be confinement dependent [6] , [7] , [11] , [12] . At present, the behaviour of interfacial water viscosity for confining surfaces with different degree of wettabilities (and different slip lengths) is unknown, thus a priori we do not know . Equation (3) indicates that the measured viscous forces on different surfaces depend on two related but distinguished phenomena: the intrinsic viscosity of nanoconfined water, which may change depending on the confining surfaces, and the slippage of water at the solid surface interface, which is already known to depend on properties such as the contact angle [18] . As, according to a previous study [19] , the slip length of hydrophilic mica is almost zero, we can assume that the viscous force measured on mica is indeed F shear b =0 ( d ) and the viscosity is . Equation (3) together with the viscous shear forces measured on mica is then used to fit the viscous forces measured on all the other surfaces with unknown . As the initial working hypothesis we have assumed that for every surface, d , the viscosity remains the same as for mica, , and we have fit all the shear viscous forces for the different surfaces with the equation: leaving b as a free-fitting parameter, to be compared with data measured or calculated in literature with different methods [18] , [19] , [20] , [21] . The fitting process is illustrated in Fig. 3 , where the experimental F shear ( d ) curves measured on partially hydrophobic HOPG, DLC, GO ( Fig. 3b–d ) and Si are fitted using the viscous force curve acquired on hydrophilic mica ( Fig. 3a ) between d ≈0.3 and 3 nm as the zero slippage viscous curve. 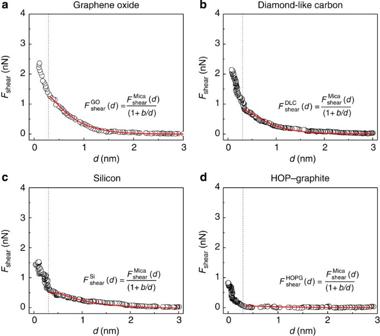Figure 3: How slip can explain the measured apparent viscosity. The lateral forces experienced by a tip approaching (a) GO, (b) DLC, (c) Si and (d) HOPG in water. The solid red lines ina–dare the fitted curves obtained by equation (4), where the only free-fitting parameter is the slip length. The coefficient of determination,R, and the reducedχ2are determined using the Levanburg–Marquette algorithm. The obtainedRis found to be 1.0 for GO, 0.99 for DLC, 0.96 for silicon and 0.4 for HOPG, whereas the reducedχ2, which represents the deviations of the fitted curve from the experimental data, is always <10−3. The error bars ofbshown inFig. 4are determined from the error of averaging the lateral force curves for GO, DLC and Si. For HOPG, the error is determined from fitting using different ranges fromd≈0.3 nm tod=3 nm. Figure 3: How slip can explain the measured apparent viscosity. The lateral forces experienced by a tip approaching ( a ) GO, ( b ) DLC, ( c ) Si and ( d ) HOPG in water. The solid red lines in a – d are the fitted curves obtained by equation (4), where the only free-fitting parameter is the slip length. The coefficient of determination, R , and the reduced χ 2 are determined using the Levanburg–Marquette algorithm. The obtained R is found to be 1.0 for GO, 0.99 for DLC, 0.96 for silicon and 0.4 for HOPG, whereas the reduced χ 2 , which represents the deviations of the fitted curve from the experimental data, is always <10 −3 . The error bars of b shown in Fig. 4 are determined from the error of averaging the lateral force curves for GO, DLC and Si. For HOPG, the error is determined from fitting using different ranges from d ≈0.3 nm to d =3 nm. Full size image The values of slip length obtained from this fitting procedure are the following: b =0.24±0.38, 0.55±1.37, 1.0±1.7 and 12.0±3.3 nm for GO, DLC, Si and HOPG, respectively. These slip-length values are then plotted as a function of the static contact angle of the corresponding surface as shown in Fig. 4a . First, these values are in good agreement with existing experimental or theoretical values found in literature [18] , [20] , [21] , [22] , [23] (see Supplementary Table S3 ). Second, the good superposition of the fitting curves with the experimental data points confirms that equation (4) is able to capture the physics behind the different observed viscous behaviours, demonstrating that the striking variations in the viscous forces at the interface are indeed related to different water slippages at the interface, while the intrinsic viscosity of nanoconfined water remains the same, independently of surface hydrophilicity at any confinement d . 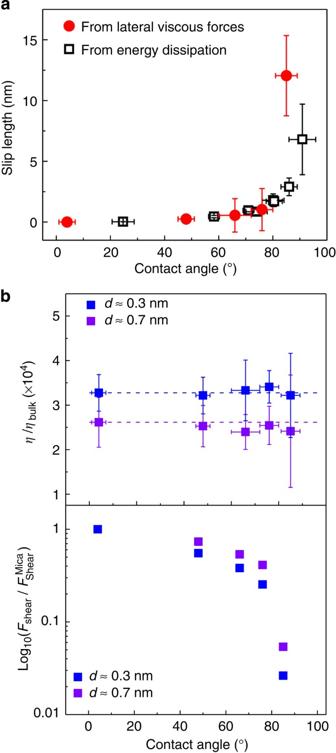Figure 4: Slip, viscosity and shear viscous force as a function of wettability. (a) Slip lengthbas a function of contact angle, wherebis extracted from the fitting curves illustrated inFig. 3(filled circles) and from the tip energy dissipation (open squares) measured during dynamic-mode AFM imaging in water. The vertical error bars indicate experimental error in these measurements, whereas the horizontal ones are obtained from the contact angle measurements. (b)η/ηbulkratio (top) andFshear/FshearMicaratio (bottom) as a function of the water contact angle of the investigated surfaces atd≈0.3 nm and 0.7 nm. Figure 4b shows for d ≈0.3 and 0.7 nm the measured and as a function of the static contact angle of the corresponding surface, where is the viscosity of bulk water at room temperature and being the viscosity of water confined (at d confinement) between a tip and a surface with the slip length b . Figure 4: Slip, viscosity and shear viscous force as a function of wettability. ( a ) Slip length b as a function of contact angle, where b is extracted from the fitting curves illustrated in Fig. 3 (filled circles) and from the tip energy dissipation (open squares) measured during dynamic-mode AFM imaging in water. The vertical error bars indicate experimental error in these measurements, whereas the horizontal ones are obtained from the contact angle measurements. ( b ) η / η bulk ratio (top) and F shear / F shear Mica ratio (bottom) as a function of the water contact angle of the investigated surfaces at d ≈0.3 nm and 0.7 nm. Full size image AFM energy dissipation measurements To prove the generality of our conclusions, we performed AFM experiments with a tip oscillating perpendicularly to a surface, in the standard configuration used in non-contact, dynamic-mode AFM. We then recorded the energy dissipation, E T , due to viscous losses as the tip oscillates in water close to a variety of solid surfaces (see Methods part and Supplementary Note 3 ). Previous work has shown that such losses are correlated with the static contact angle of the surfaces [24] , [25] , but the physical origin of this link has to date not been explained. Motivated by our new understanding, we argue that the average energy costs associated with the subsequent approach and retraction of a tip vertically oscillating within ~1 nm from a surface (interface) can be explained by water slippage, as it is proportional to the viscous forces at that interface, as modelled in equation (4): where E T b =0 is the energy dissipation measured on mica and E T b is the energy dissipation measured on a surface with a given slip length and contact angle. We then obtain the slip length as a function of the contact angle of the surface over which the energy dissipation is measured by using equation (5) in the form of , for d =1 nm. The results, presented as open squares in the Fig. 4a along with the values of b versus contact angle as found from the fitting of the shear viscous forces shown in Fig. 3 , display a clear agreement between the viscous force shearing experiments and the compressive dissipation experiments, demonstrating that in both cases the water slip length is at the origin of the wettability-dependent viscous dissipation. Significantly, these results also provide a new framework for interpreting AFM experiments in water. Furthermore, in Fig. 5 we plotted for d =1 nm the ratio between the viscous force on an arbitrary surface and on mica, as well as the ratio of the compressive energy dissipation on an arbitrary surface and on mica, as a function of the slip length of the corresponding surface. These ratios fall on a single master curve equal to d /( b + d ). 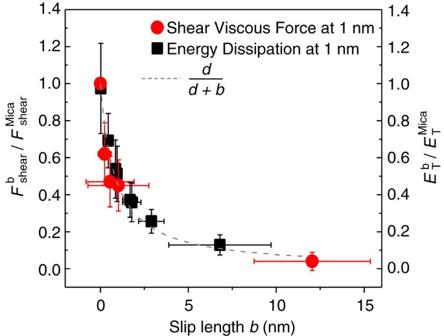Figure 5: Shear viscous forces and energy dissipation versus slip length. Water interfacial viscous forces ratios (filled circles) and energy dissipation (filled squares) ratios as a function of the slip length ford=1 nm, wherebis extracted, respectively, from the fitting curves illustrated inFig. 3using equation (4), and from the energy dissipation measured during dynamic-mode AFM imaging in water by using equation (5). These ratios fall on the master curve equal tod/(b+d). The vertical error bars are obtained from multiple measurements ofFshearandET, whereas the horizontal error bars are determined from the fitting procedure illustrated inFig. 3. Figure 5: Shear viscous forces and energy dissipation versus slip length. Water interfacial viscous forces ratios (filled circles) and energy dissipation (filled squares) ratios as a function of the slip length for d =1 nm, where b is extracted, respectively, from the fitting curves illustrated in Fig. 3 using equation (4), and from the energy dissipation measured during dynamic-mode AFM imaging in water by using equation (5). These ratios fall on the master curve equal to d /( b + d ). The vertical error bars are obtained from multiple measurements of F shear and E T , whereas the horizontal error bars are determined from the fitting procedure illustrated in Fig. 3 . Full size image Figures 4 and 5 show the main conclusive results of this study, namely the relationship between water interfacial viscous forces, energy dissipation and slippage at that interface. In particular, our results demonstrate that interfacial viscous forces and the dissipated energy during compression in nanoconfined water can decrease of up to two orders of magnitude due to water slippage, whereas the intrinsic viscosity (top panel in Fig. 4b ) remains extremely high compared with bulk water and approximately independent of surface hydrophilicity for every confinement size, and for the surfaces here investigated. The origin of such a large viscosity of nanoconfined water is not completely understood. Certainly it is important to remark that we are dealing with only three to four water atomic layers where water may undergo structural changes such as layering effects, a slow-down of water dynamics due to confinement or nano-jamming effects. We remark that although these results are possibly limited to surfaces that are ultra-smooth and with hydrophobicity below 90°, the conclusions provide a new general understanding of interfacial phenomena, which may have an impact in a wide range of studies and applications. In summary, we have studied water interfacial viscosity on substrates with different wettability. Our results demonstrate that boundary viscous forces are related to slippage processes, which in turn can depend on the wettability of the interfacial surface. A modified form of the Newtonian definition of viscosity, which takes the fluid slip into account, is successfully used to explain that the decrease of the interfacial viscous forces with increasing hydrophobicity is due to a respective increase in slip length, whereas the intrinsic viscosity of nanoconfined water remains the same for all the surfaces investigated here, at any confinement size. The same model is also used to quantitatively explain the so-far unclear relationship between surface wettability and energy dissipation in dynamic AFM experiments. Beyond the reign of water, this new understanding of the interplay between interfacial viscosity, wettability and boundary slip might explain the change in glass transition temperature of very thin polymer films as a function of the polymer wettability of the substrate [26] . Finally, this work opens up new strategies to investigate the hydration layers in complex systems, such as proteins [1] and cytoskeletal filaments [27] . Water purity DIUF water was purchased from Fischer Scientific, and the purity was confirmed with an AB30 Conductivity Meter (Fischer Scientific). The measurement indicated a resistance of 18 MΩ, corresponding to an ion concentration of <0.04 p.p.m. Viscous force measurements The lateral viscous force experiments were performed in DIUF water with an AFM (Picoplus 5500, Agilent) at room temperature. A silicon AFM cantilever with typical normal and lateral spring constants equal to k N ≈3 to 5 N m −1 and k T ≈50 to 120 N m −1 , respectively, are used. The calibration is discussed in Supplementary Note 4 and Supplementary Fig. S2 . The tip radius is ~40 nm, as measured by scanning electron microscope (JOEL JSM-5910) imaging after each experiment. The influence of the tip shape and radius on the measured lateral viscous force is discussed in Supplementary Note 5 . The AFM tip approaches the hard solid surface at a vertical speed of 0.2 nm s −1 . The shearing frequency, 1 kHz, and amplitude, 0.9 nm, are controlled by a lock-in amplifier. See also refs 6 , 7 . For each surface, several lateral and normal force versus separation d curves were obtained ( Supplementary Fig. S3 ). These force curves are averaged as shown in Fig. 2 . Muscovite mica and HOPG (both from SPI Supplies, West Chester, PA) were prepared for experiments via the tape-refresh method in ambient conditions. The mica and HOPG surface were blown with ultrapure compressed nitrogen gas to eliminate any surface debris, after which it was immediately inserted into the liquid cell for lateral force measurements. GO was synthesized by oxidation of epitaxial graphene using the Hummers method [28] , [29] . Si and DLC surfaces, grown by Pulsed Laser Deposition [30] in vacuum, were cleaned by rinsing with ethanol (95%), followed by sonication in ethanol and dried with compressed nitrogen gas. The same procedure, that is, rinse/sonication was then repeated with isopropyl alcohol and DIUF water. The N-doped (100) silicon substrates (University Wafer, South Boston, MA) was cleaned by rinsing with DIUF water followed by sonication in DIUF water. The same procedure, that is, rinse/sonication was then repeated with ethanol (95%), isopropyl alcohol and DIUF water again and then blown dried with compressed nitrogen gas. The contact angle was measured with a Contact Angle Meter (Phoenix 150, SEO). Energy dissipation measurements Measurements of the local energy dissipation were performed with a Multimode Nanoscope IIIa AFM (Digital Instruments) equipped with an external lock-in amplifier. The AFM was operated in amplitude-modulation mode with the cantilever driven close to its resonance in water. The tip and sample were fully immersed in ultrapure water. While imaging, the system was adjusted so as to ensure that most of the tip oscillation (and damping) occurs within the interfacial water at the surface of the solid. This is typically achieved using vibration amplitudes of ~1 nm and ‘soft’ scanning setpoints [24] . The tip vibration amplitude and phase (phase lag with the driving vibration) were acquired for each point (pixel) of the imaged sample. Knowing the cantilever stiffness and Q -factor (calculated from the cantilever thermal spectrum [31] ), the tip local energy dissipation is calculated using the simple harmonic oscillator formalism [32] . The energy dissipation values presented in Figs 4 and 5 represent averages of the calculated local energy dissipation over areas covering several tens of nanometre squares. We investigated energy dissipation on mica, silicon oxide, aluminum oxide, strontium titanate, optical grad calcite, silicon carbide, titanium dioxide, fluorite and HOPG, with contact angles of <20°, 24°, 58.3°, 71°, 74°, 80.1°, 80.5°, 86° and 90.9°, respectively. Mica surfaces (SPI Supplies) were cleaved immediately before use. Optical grade calcite (Iceland Spar) and fluorite (from Hunan, China) samples were cleaved with a razor blade along the desired plane ([1014] for calcite and [111] for fluorite) and subsequently incubated for several days in ultrapure water (18.2 MΩ, Millipore, Billerica, MA, USA) to allow the samples to equilibrate with the solution. All the other crystals, namely silicon carbide, aluminum oxide, strontium titanate, titanium dioxide and silicon oxide were purchased from MTI Corp. (Richmond, CA, USA), and were already Epitax Ready-polished according a predefined crystalline direction. The crystals were cleaned by successive sonication in dimethylsulphoxide, ethanol, acetone, and ultrapure water. Mitigation of errors Nanoscale measurements are inherently sensitive to surface imperfection such as nanoscale singularities and contamination. Here we take several steps to mitigate these problems. First, we used atomically smooth surfaces, such as single crystals, with consistent surface cleaning procedures and conducted the AFM measurements in a clean and controlled environment. Possible contaminations (for example, due to hydrocarbon molecules) tend to induce dramatic effects on the measurements, which can be unambiguously discarded. Furthermore, all the measurements were repeated several times on different locations of each sample. Finally, complementary nanoscale approaches were conducted independently in two different laboratories, always yielding the same general trend, which can be explained by our simple model. How to cite this article: Ortiz-Young, D. et al. The interplay between apparent viscosity and wettability in nanoconfined water. Nat. Commun. 4:2482 doi: 10.1038/ncomms3482 (2013).